Dynamic evolution of precise regulatory encodings creates the clustered site signature of enhancers Concentration gradients of morphogenic proteins pattern the embryonic axes of Drosophila by activating different genes at different concentrations. The neurogenic ectoderm enhancers (NEEs) activate different genes at different threshold levels of the Dorsal (Dl) morphogen, which patterns the dorsal/ventral axis. NEEs share a unique arrangement of highly constrained DNA-binding sites for Dl, Twist (Twi), Snail (Sna) and Suppressor of Hairless (Su(H)), and encode the threshold variable in the precise length of DNA that separates one well-defined Dl element from a Twi element. However, NEEs also possess dense clusters of variant Dl sites. Here, we show that these increasingly variant sites are eclipsed relic elements, which were superseded by more recently evolved threshold encodings. Given the divergence in egg size during Drosophila lineage evolution, the observed characteristic clusters of divergent sites indicate a history of frequent selection for changes in threshold responses to the Dl morphogen gradient and confirm the NEE structure/function model. How genetic information is encoded in DNA is a central question in biology. Much of this information is encoded during the natural selection of mutational changes within regulatory DNA sequences, which specify the conditions under which a gene product is made by a cell [1] , [2] , [3] , [4] , [5] , [6] , [7] , [8] , [9] , [10] . However, identification of functional regulatory changes is difficult because, unlike the precise protein-encoding scheme, few regulatory-encoding schemes have been identified. Identifying such regulatory-encoding schemes by studying the sequences of cis -regulatory modules (CRMs) would advance many areas of biological investigation. CRMs, such as the developmental enhancers that read classical morphogen concentration gradients [11] , are ideal subjects in decoding regulatory DNA sequences and their functional features. Different enhancers targeted by the same transcription factor (TF) each respond to their own unique threshold concentration of TF. These DNAs can be compared to identify potential variables that encode this concentration threshold setting. Two such systems of morphogen-responsive enhancers are those that read the Bicoid and Dorsal (Dl) morphogen concentration gradients, which pattern the anterior/posterior (A/P) and dorsal/ventral axes of the Drosophila embryo, respectively [12] , [13] , [14] , [15] , [16] , [17] , [18] , [19] , [20] , [21] , [22] , [23] . Similar to many enhancers, these DNAs contain homotypic clusters of variant sites related to the binding preferences of their respective TFs. Such site clustering has prompted several complex models that integrate site number, quality and density parameters to model known enhancers and identify new enhancers [24] , [25] , [26] , [27] , [28] . However, little progress has been made in integrating these variables into a model that predicts their precise threshold-specific responses. The neurogenic ectoderm enhancers (NEEs) represent an unprecedented example corpus of CRMs that have been evolving independently at multiple loci throughout the Drosophila genus in order to encode appropriate threshold responses at the lower ranges of the Dl morphogen gradient [6] , [29] . Furthermore, this genus has experienced tremendous lineage-specific, ecological specialization for different egg-laying habitats. Among other changes, this diversification involved changes in egg size and timing of embryogenesis. Such changes are expected to have necessitated compensatory changes in the shapes of morphogen gradients [23] and the sequences of their threshold-encoding target enhancers [6] . NEEs in any genome are identifiable through a unique arrangement of cis -regulatory elements that bind Dl, Twist (Twi), Snail (Sna) and Suppressor of Hairless (Su(H)) [29] . The NEE at the vnd locus, or NEE vnd , is conserved in Drosophila and mosquitos [29] . Thus, it was present in the latest common ancestor of dipterans ∼ 240 to 270 million years ago [30] , [31] , [32] . NEE vnd is part of a canonical set of four NEEs that occur across the Drosophila genus and includes NEEs at the rho , brk and vn loci. A more recently evolved member of this enhancer class, NEE sog , occurs upstream of the sog locus of the melanogaster subgroup, which began diverging ∼ 20 million years ago [6] . Thus, altogether, NEE-type regulatory sequences have been evolving at various unrelated loci during the last ∼ 250 million years. In the NEEs from D. melanogaster , D. pseudoobscura and D. virilis , we found that (i) the threshold concentration is encoded in the precise length of a spacer element, which separates well-defined Twi- and Dl-binding sites: 5′-CACATGT-3′ (polarized), 3–18 bp spacer, 5′-SGGAAABYCCM-3′ (IUPAC consensus motif occurs in either orientation), and (ii) these cis -regulatory adjustments have been performed at all NEEs across a given genome, consistent with their co-evolution to a common change in trans [6] . However, although we identified the unique functional spacer element and its role in encoding precise threshold responses to Dl, we had yet to address the spacer's full functional range and the function of the many other variant, loosely organized Dl-binding sites, which constitute the homotypic site clusters observed at these enhancers. As such, it was not clear whether these additional variant sites were necessary and/or sufficient for modulating the threshold-specific response to the Dl gradient, participating in activation or repression, or controlling any other regulatory function. Here, we study NEEs from the D. ananassae and D. willistoni genomes, which may contain evolutionary signatures that are absent in the relatively compact genomes of the melanogaster subgroup. These results reveal information about the process and frequency by which compensatory threshold changes occur, and support a novel molecular evolutionary model of enhancer function and homotypic site cluster formation. There are three interdependent components of the model. First, threshold evolution is facilitated by a molecular-encoding scheme that requires only a single pair of adjacent Dl and Twi elements, whose palindromic nature allows the threshold setting to be easily changed by acquisition of a new partner site. This process produces a byproduct in the form of relic elements, which constitute the observed homotypic site clusters. Second, all new spacer variants are produced by expansion and contraction mutations of a specific satellite repeat sequence that functions as the Twi-binding element. Third, the magnitude of relic element accumulation in the oldest enhancers is such that subsequent selection for replacement sites for any TF is highly biased by the background relic sequence composition of the enhancer. Thus, functional elements acquire a non-functional patina, as the enhancer ages over millions of years of adaptive threshold maintenance. Altogether, the resulting model simplifies explanation of an increasing amount of anomalous data about enhancers, including rapid non-functional divergence in the sequence components of homotypic site clusters [33] , enrichment for site clustering in embryonic enhancers relative to other tissues that also employ morphogen gradients [34] and the threshold-independent variance of binding site quality in many well-studied embryonic enhancers [35] . A characteristic site cluster signature marks older NEEs We find that a novel signature of clustered sites is associated with NEEs that are conserved across five divergent Drosophila species, including three species with large, uncompacted genomes ( Fig. 1a ). This clustered site signature bears a distinct relationship to the previously reported specialized sites of NEEs [6] , [29] . This signature marks the oldest NEEs with a continuum of sequences that begins with one well-defined Dl-binding element that is closest to the Twi-binding element and continues with an increasing number of more divergent sequence fragments related to this specific Dl-binding element ( Fig. 1b ). The compositional range of these increasingly fainter sites extends beyond sequences considered to be functional low-affinity Dl-binding sites. We refer to these fainter, 'ghost' sequences as relic elements. 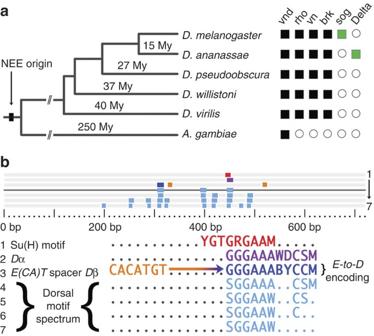Figure 1: Organization of specialized sites within Dl relic site clusters. (a) Phylogeny ofDrosophilawith table of canonical NEEs. A certain signature of clustered relic sites characterizes the canonical NEEs, which are found in four unrelated gene loci acrossDrosophila(black boxes). Newer lineage-specific NEEs are found in other loci (green boxes). Open circles represent an absence of an NEE-type sequence at the locus. (b) Features of a typical relic site cluster in a canonical NEE. Canonical NEEs possess the three specialized sites: a Su(H)-binding site (red motif) that overlapsDα motif (purple motif), the linkedE(CA)TandDβ motifs (orange and blue motifs, respectively) and the Dl variant relic sites, which can be visualized with a spectrum of increasingly degenerate versions of theDβ motif (light blue motifs). Each motif-matching sequence is visualized in a separate numbered track (1–7) at the top and described in more detail below. This particular enhancer corresponds to thevndNEE ofD. melanogaster. The motif sequences in all the figures and text are written according to IUPAC DNA convention: S=[CG], W=[AT], R=[AG], Y=[CT], K=[GT], M=[AC], B=[CGT], D=[AGT], H=[ACT], V=[ACT], N=[ACGT], where nucleotides in brackets are equivalent.A. gambiae,Anopheles gambiae; My, million years. Figure 1: Organization of specialized sites within Dl relic site clusters. ( a ) Phylogeny of Drosophila with table of canonical NEEs. A certain signature of clustered relic sites characterizes the canonical NEEs, which are found in four unrelated gene loci across Drosophila (black boxes). Newer lineage-specific NEEs are found in other loci (green boxes). Open circles represent an absence of an NEE-type sequence at the locus. ( b ) Features of a typical relic site cluster in a canonical NEE. Canonical NEEs possess the three specialized sites: a Su(H)-binding site (red motif) that overlaps D α motif (purple motif), the linked E(CA)T and D β motifs (orange and blue motifs, respectively) and the Dl variant relic sites, which can be visualized with a spectrum of increasingly degenerate versions of the D β motif (light blue motifs). Each motif-matching sequence is visualized in a separate numbered track (1–7) at the top and described in more detail below. This particular enhancer corresponds to the vnd NEE of D. melanogaster . The motif sequences in all the figures and text are written according to IUPAC DNA convention: S=[CG], W=[AT], R=[AG], Y=[CT], K=[GT], M=[AC], B=[CGT], D=[AGT], H=[ACT], V=[ACT], N=[ACGT], where nucleotides in brackets are equivalent. A. gambiae , Anopheles gambiae ; My, million years. Full size image We find a definitive property distinguishing numerous relic elements from the functional elements, which we have called specialized elements because of how they are detected [6] , [29] . Although the functional elements fit NEE-specific TF-binding motifs that are highly conserved across the entire genus, the clustered relic elements can only be described by increasingly degenerate versions of the motifs for the functional elements. In mathematical terms, there is no sequence motif that can identify a unique site from among the relic elements at each NEE. This distinction provides a method for distinguishing functional parent elements from their clustered relic counterparts. Three site motifs are relevant to our experiments and concluding model of relic element production, namely, SUH / D α, D β and E(CA)T ( Fig. 1b ). These motifs are specialized versions of general binding motifs for Su(H), Dl and Twi and Sna, respectively. The motif D α partially overlaps with the overly determined Su(H)-binding site SUH , whereas the Dl-binding motif D β is located within ∼ 20 bp of the E(CA)T element, closer than any other Dl-binding site variant. The E(CA)T element is a specialized CA-core E-box with an additional T, that is, 5′-CACATGT-3′, and its slight palindromic asymmetry points downstream to D β, which is also palindromic but not polarized. We will refer to the three arranged elements of the polarized E(CA)T site, the threshold-setting spacer and an unpolarized D β site, as an E-to-D encoding of a specific threshold response. D. willistoni NEEs are enriched in relic sites We analysed the D. willistoni genome, which is the largest assembled Drosophila genome (224 Mb) [36] , and an early branch of the Sophophora subgenus, which also includes the compacted genomes of the melanogaster subgroup. We identify only four canonical NEEs when we search the entire D. willistoni genome assembly sequence for all 800 bp sequences containing any arrangement of the three motifs SUH / D α, D β and E(CA)T . Despite significant sequence divergence, these NEE sequences conform to the aforementioned syntactical rules. These NEE-bearing loci are expressed in the neurogenic ectoderm of D. willistoni embryos, as shown by whole-mount in situ hybridization, with anti-sense probes against the D. willistoni transcripts ( Fig. 2a–d ). 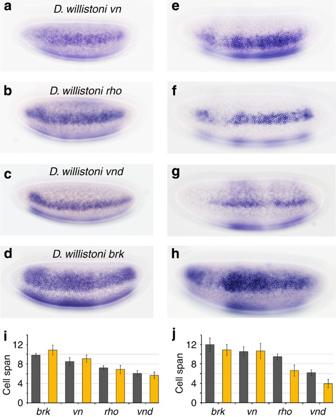Figure 2: Functional NEEs fromD. willistoni. (a–d) Endogenousin situhybridization experiments for NEE-bearing loci inD. willistonistage 5(2) embryos forvn(a),rho(b),vnd(c) andbrk(d). (e–h) NEE-drivenlacZ in situhybridization experiments forD. willistoniNEEs. Shown are lateral stripe expression patterns that are typical of multiple transgenicD. melanogasterlines made with theD. willistoniNEEs fromvn(e),rho(f),vnd(g) andbrk(h). Embryos in all figures are depicted with anterior pole to the left and dorsal side on top. (i) Graph showing the number of cells (nuclei) spanned by the lateral stripe of expression of orthologous NEE-bearing genes fromD. melanogaster(dark grey) andD. willistoni(orange). (j) Graph showing the number of cells (nuclei) spanned by thelacZexpression pattern driven by various NEEs.D. willistoniNEEs (orange) drive identical (brkandvn) or slightly reduced (rhoandvnd) expression patterns relative to theD. melanogasterorthologs (dark grey). Error bars represent ±1 s.d. and are obtained by counting number of nuclei spanned at 50% egg length for several stage 5(2) embryos from at least three independent transgenic lines. Figure 2: Functional NEEs from D. willistoni . ( a – d ) Endogenous in situ hybridization experiments for NEE-bearing loci in D. willistoni stage 5(2) embryos for vn ( a ), rho ( b ), vnd ( c ) and brk ( d ). ( e – h ) NEE-driven lacZ in situ hybridization experiments for D. willistoni NEEs. Shown are lateral stripe expression patterns that are typical of multiple transgenic D. melanogaster lines made with the D. willistoni NEEs from vn ( e ), rho ( f ), vnd ( g ) and brk ( h ). Embryos in all figures are depicted with anterior pole to the left and dorsal side on top. ( i ) Graph showing the number of cells (nuclei) spanned by the lateral stripe of expression of orthologous NEE-bearing genes from D. melanogaster (dark grey) and D. willistoni (orange). ( j ) Graph showing the number of cells (nuclei) spanned by the lacZ expression pattern driven by various NEEs. D. willistoni NEEs (orange) drive identical ( brk and vn ) or slightly reduced ( rho and vnd ) expression patterns relative to the D. melanogaster orthologs (dark grey). Error bars represent ±1 s.d. and are obtained by counting number of nuclei spanned at 50% egg length for several stage 5(2) embryos from at least three independent transgenic lines. Full size image Using PCR, we cloned DNA fragments encompassing the four distinct NEE sequences of D. willistoni and individually tested them for enhancer activity on a lacZ reporter gene stably integrated into multiple independent lines of D. melanogaster . Whole-mount in situ hybridization of transgenic stage 4 to stage 5 embryos with an anti-sense lacZ probe shows that the D. willistoni enhancers drive robust lateral ectodermal expression in D. melanogaster embryos ( Fig. 2e–h ), although with slightly narrower expression patterns than their D. melanogaster orthologs ( Fig. 2i–j ). Using a spectrum of increasingly degenerate Dl-binding motifs, we find Dl relic site clusters in the NEEs of D. willistoni ( Supplementary Figs S1 , S2 ). We find a D α motif that identifies within each NEE a single Dl variant site that overlaps the Su(H)-binding site ( Supplementary Fig. S1 ). We find a D β motif that identifies within each NEE the closest variant Dl site adjacent to E(CA)T ( Supplementary Fig. S2 ). These D α and D β motifs describe separate unique sites within each enhancer. However, unlike D α, the D β consensus motif for the NEEs of D. willistoni is nearly identical with the corresponding motif in other lineages ( Supplementary Table S1 ). We also find that the Dl relic element clusters of NEEs from D. willistoni are enriched in lengthy CA-satellite tracts ( Supplementary Fig. S3 ). In fact, specific CA-dinucleotide repeats are associated with specific constituents of Dl relic elements. Conversely, almost all constituent sites of Dl relic elements are associated with prominent CA-satellite tracts. For example, the NEE vn of D. willistoni has expanded CA-satellite tracts coordinated to divergent D β elements at ∼ 340 to 400 bp and again at ∼ 580 to 630 bp, whereas the D. willistoni NEE rho also has expanded CA-satellite tracts coordinated to divergent D β elements at ∼ 130 to 150 bp and again at ∼ 270 to 290 bp. Last, the NEE vnd sequence, which is at least ∼ 250 million years old, is characterized by the greatest number of lengthy CA-satellite tracts ( Fig. 3a ). Given that the E(CA)T sequence, 5′-CACATGT-3′, is composed entirely of CA-dinucleotide repeats, these results suggest that these CA-dinucleotide repeats are the E(CA)T motif's relic counterparts, and possibly that runaway tract expansions persist in lineages with uncompacted genomes. 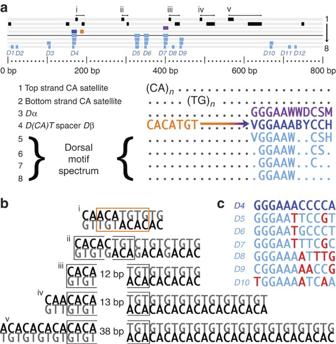Figure 3: ThevndNEE fromD. willistoniis enriched in palindromic CA satellite. (a) Graph of the relic site cluster of thevndNEE sequence from the relatively uncompactedD. willistonigenome. Each motif-matching sequence is visualized in a separate numbered track (1–8) at the top and described in more detail below. Similar to other canonical NEEs fromD. willistoni, this sequence contains lengthy, split, palindromic CA-satellite tracts (roman numerals) on both strands, as visualized by matches to the short CA-satellite motifs 5′-CACA-3′ or 5′-ACAC-3′ (tracks no. 1 and no. 2). Inferred Dl relic sites as visualized by the Dl motif spectrum are visualized on the bottom tracks and numbered for reference underneath the bottom-most track (D1–D12). (b) The exact sequences of the palindromic CA-satellite tracts (i–v). CA satellite or its fragments are shown in black and the intact or splitE(CA)Tmotifs indicated with orange or split grey boxes, respectively. (c) A list of the Dl variant sites numbered in panela.Dβ is shown dark blue, whereas relic Dl sites are shown in light blue and positions of divergence fromDβ in red. Figure 3: The vnd NEE from D. willistoni is enriched in palindromic CA satellite. ( a ) Graph of the relic site cluster of the vnd NEE sequence from the relatively uncompacted D. willistoni genome. Each motif-matching sequence is visualized in a separate numbered track (1–8) at the top and described in more detail below. Similar to other canonical NEEs from D. willistoni , this sequence contains lengthy, split, palindromic CA-satellite tracts (roman numerals) on both strands, as visualized by matches to the short CA-satellite motifs 5′-CACA-3′ or 5′-ACAC-3′ (tracks no. 1 and no. 2). Inferred Dl relic sites as visualized by the Dl motif spectrum are visualized on the bottom tracks and numbered for reference underneath the bottom-most track ( D1–D12 ). ( b ) The exact sequences of the palindromic CA-satellite tracts (i–v). CA satellite or its fragments are shown in black and the intact or split E(CA)T motifs indicated with orange or split grey boxes, respectively. ( c ) A list of the Dl variant sites numbered in panel a . D β is shown dark blue, whereas relic Dl sites are shown in light blue and positions of divergence from D β in red. Full size image Homotypic site clusters are non-functional relic sequences In the NEE vnd module of D. willistoni , we detect the unambiguous inactivation of one of two E-to-D encodings still present in orthologous sequences from D. melanogaster , D. pseudoobscura and D. virilis ( Fig. 3a ). In D. melanogaster , the first E-to-D encoding has a tighter spacer compared with the second, distantly spaced E-to-D encoding. Although the E(CA)T element of this second divergent encoding is intact in other species, in D. willistoni it is expanded on both sides and split apart ( Fig. 3a , inverted CA-satellite palindromic pair no. iv). This NEE vnd of D. willistoni is marked by several other increasingly lengthy palindromic tracts, of which the intact but also expanded E(CA)T site is the leftmost site in the series ( Fig. 3b ). These expanded CA-satellite palindromes are associated with Dl variant sequences that are increasingly divergent from the D β motif ( Fig. 3c ). Although the D. willistoni NEE vnd sequence has lost an intact E(CA)T site at the second E-to-D encoding, we did not know whether this encoding functions in species in which this element is still intact. We therefore tested in transgenic reporter assays two different fragments contained within our 'full-length' 949 bp NEE vnd sequence from D. melanogaster ( Fig. 4a ). We tested an upstream 300 bp fragment that contains a 10 bp E-to-D spacer, and a separate downstream 266 bp fragment that contains the longer 20 bp E-to-D spacer. Both fragments overlap in the middle of the enhancer, which contains the SUH / D α supersite. We find that the upstream 300 bp fragment drives reporter gene expression at the same threshold setting as the full-length fragment ( Fig. 4b–c ). In contrast, the downstream 266 bp fragment does not drive reporter gene expression in a lateral stripe of any measurable width, although faint patches of sporadic ventral neuroectodermal expression are seen in a few rare embryos ( Fig. 4d–e ). Thus, the upstream E-to-D encoding, which is tightly spaced, is sufficient for the complete threshold response, whereas the second E-to-D encoding, which is expansively spaced to a D β variant, is both non-functional by itself and dispensable to neighbouring functional elements. This relic D β sequence appears to be decaying, as it has diverged from the genus-wide D β consensus ( Fig. 4f ). These results indicate that the divergent Dl-binding sites and their associated CA-satellite tracts are non-functional relic E-to-D encodings, which are frequently replaced, or superseded and deprecated, by adaptive sweeps of threshold variants during lineage evolution. 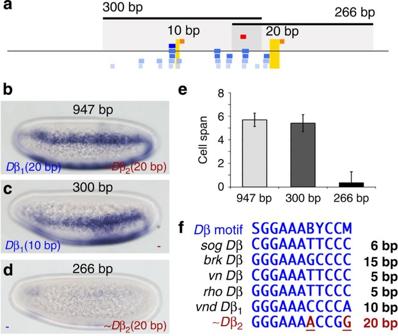Figure 4: RelicE-to-Dencodings become inactivated by mutations in elements or spacing. (a) Diagram showing two assayed sub-fragments from the 947 bpD. melanogaster vndNEE. A 300 bp sub-fragment contains anE-to-Dencoding coordinated by a 10 bp spacer (narrow yellow column). A separate, but overlapping, 266 bp fragment contains a possibleE-to-Dencoding coordinated by a 20 bp spacer (wide yellow column). All sites matching the motifs for Su(H) (red),E(CA)T(orange) andDβ (blue), and aDβ motif spectrum (increasingly lighter shades of blue) are shown. (b) Typicalin situ lacZexpression pattern given by the parent 947 bpvndNEE fragment. (c) Typicalin situ lacZexpression pattern given by the 300 bpvndNEE sub-fragment. (d)In situ lacZexpression pattern given by the 266 bpvndNEE sub-fragment, as seen in a rare embryo with faint staining. Most embryos stained from these reporter lines lack any expression. (e) Quantification of the stripe width over several embryos for each construct depicted in panelsa–d. Error bars represent ±1 s.d., as derived from three independent replicates of at least 20 embryos for each construct. (f) A comparison ofDβ sequences fromD. melanogasterNEEs, including the two closest matches from thevndNEE. Divergence in sequence or its adjacent spacer length toE(CA)Tis depicted in dark red. Figure 4: Relic E-to-D encodings become inactivated by mutations in elements or spacing. ( a ) Diagram showing two assayed sub-fragments from the 947 bp D. melanogaster vnd NEE. A 300 bp sub-fragment contains an E-to-D encoding coordinated by a 10 bp spacer (narrow yellow column). A separate, but overlapping, 266 bp fragment contains a possible E-to-D encoding coordinated by a 20 bp spacer (wide yellow column). All sites matching the motifs for Su(H) (red), E(CA)T (orange) and D β (blue), and a D β motif spectrum (increasingly lighter shades of blue) are shown. ( b ) Typical in situ lacZ expression pattern given by the parent 947 bp vnd NEE fragment. ( c ) Typical in situ lacZ expression pattern given by the 300 bp vnd NEE sub-fragment. ( d ) In situ lacZ expression pattern given by the 266 bp vnd NEE sub-fragment, as seen in a rare embryo with faint staining. Most embryos stained from these reporter lines lack any expression. ( e ) Quantification of the stripe width over several embryos for each construct depicted in panels a – d . Error bars represent ±1 s.d., as derived from three independent replicates of at least 20 embryos for each construct. ( f ) A comparison of D β sequences from D. melanogaster NEEs, including the two closest matches from the vnd NEE. Divergence in sequence or its adjacent spacer length to E(CA)T is depicted in dark red. Full size image Thresholds are sourced from a single mutational mechanism Although new threshold encodings can occur by selection of spacer length variants defined by existing elements, they can also occur by selection of new replacement elements that define new spacers. Three inherent features of E-to-D encodings increase the capacity for selective amplification of these replacement encodings. One feature is the palindromic nature of E(CA)T and D β, which allows new E-to-D encodings to arise from a single emergent site that is located on the other side of its coordinating partner element in an existing encoding ('a leapfrog'). A second feature is that the E-to-D spacer's functional range is broad and capable of producing near-optimal encodings with adaptive potential. A third feature is that a generic Twi-binding site can evolve to resemble a specific CA-dinucleotide satellite sequence, which is susceptible to repeat expansions and contractions across the Drosophila genus [37] , [38] , [39] . This third feature can accelerate the optimization of existing encodings as well as new replacement encodings by generating spacer length variants and/or new Twi-binding sites. We sought to corroborate or reject this hypothesized role of CA-satellite-repeat-induced mutation during threshold evolution. According to this idea, selection for new thresholds amplifies spacer length variants, which are predominantly produced by one specific mutational mechanism. To be consistent with our data, this hypothesis would also require that the fixation rate of synonymous mutations at a functional Twi-binding site is much less than the rate of selective sweeps for new spacer variants produced by CA-satellite-rich Twi-binding sites. We therefore aligned and compared all of the flanking sequences extending from the E(CA)T heptamer across orthologous NEEs. We find that these intact E(CA)T elements are frequently repeat-expanded beyond the core Twi-binding heptamer such that they match the general pattern given by 5′-(CA) n T(GT) m -3′, where n ≥2 and m ≥1 ( Supplementary Table S2 ). This finding supports the idea that CA-satellite instability is the source of new threshold setting spacers and possibly new Twi-binding sites as well. Alternatively, the observed constraint in the E(CA)T sequence could be partially explained as the superimposition of binding preferences for Twi and Sna. Activating Twi:Da basic helix–loop–helix heterodimers bind the YA-core E-box 5′-CAYATG-3′, whereas the mesodermal Sna repressor binds to the motif 5′-SMMCWTGYBK-3′(refs 40 , 41 ). However, selection for such a dual-functioning site should result in the motif 5′- S CACATG YBK -3′ (underlined sequence at odds with data), which we do not observe in the study of 22 different NEEs from 5 different Drosophila genomes. To address the magnitude of CA-satellite accumulation in NEEs across the genus, we computed the percentage of CA satellite in NEEs from D. melanogaster , D. pseudoobscura , D. willistoni and D. virilis relative to their genomic background levels ( Supplementary Table S3 ). We find that the NEEs are enriched relative to their genomes and that their intact E(CA)T motifs constitute only a minor fraction of this CA-repeat sequence ( Supplementary Table S3 ). These analyses show that CA satellite is enriched in NEEs above genomic background rates because of relic sites and not because of intact functional elements. To address the possibility that elevated CA-satellite composition is a feature common to developmental enhancers, we looked at several embryonic enhancers that respond to the Bicoid morphogen gradient, which patterns the A/P axis. We identified complete orthologous sequence sets for the hb embryonic enhancer [42] , the gt posterior stripe enhancer [43] , the Kr central domain enhancer [44] , [45] and the eve stripe 2 enhancer [46] from each of four genomes, namely, D. melanogaster , D. pseudoobscura , D. willistoni and D. virilis . All of these enhancers are active in the same embryonic nuclei as the NEEs and thus constitute a well-matched control group. We find that while the NEE set from any genome is enriched in CA-satellite dinucleotide and trinucleotide fragments, none of the 16 A/P enhancer sets possess the elevated CA-satellite levels that characterize canonical NEEs from these same species, even in genomes with elevated CA-satellite content ( Fig. 5a–b ). 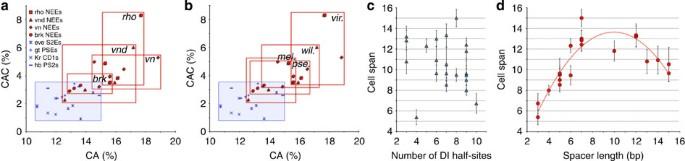Figure 5: Relic sites are non-functional and accumulate as the enhancer ages. (a) Graph showing the percentage of CA-dinucleotide and CAC-trinucleotide content of several orthologous enhancer sequences fromD. melanogaster,D. pseudoobscura,D. willistoniandD. virilis. Each window of NEE sequence is taken ±480 bp fromDβ for each species. Each window of an A/P enhancer is a 960 bp sequence centred around the Bicoid-binding site cluster. Each orthologous set of NEEs is boxed separately to visualize enrichment relative to other groups. The red boxes show the regions occupied by all data points corresponding to a single orthologous set of NEEs located at the indicated locus across many species. The blue box shows the region occupied by all data points corresponding to all A/P enhancers for all species. (b) Identical graph as in panela, except the data points are boxed by species to visualize genome-specific effects in satellite enrichment or depletion. Red boxes show the region occupied by all data points corresponding to all NEEs within a single species. Canonical A/P enhancers at theeve,gt,Krandhbloci for all four species are boxed in both panels (blue rectangular area). (c) Graph showing the number of cells spanned by thelacZexpression pattern (vertical axis), as driven by NEEs containing different numbers of Dl half-sites, 5′-SGGAAW-3′ (horizontal axis). (d) Graph showing the number of cells spanned by thelacZexpression pattern (vertical axis), as driven by NEEs characterized by differentE-to-Dspacer lengths (horizontal axis). Error bars incanddrepresent ±1 s.d., as derived from a replicate pool of 20–120 embryos for each construct. Figure 5: Relic sites are non-functional and accumulate as the enhancer ages. ( a ) Graph showing the percentage of CA-dinucleotide and CAC-trinucleotide content of several orthologous enhancer sequences from D. melanogaster , D. pseudoobscura , D. willistoni and D. virilis . Each window of NEE sequence is taken ±480 bp from D β for each species. Each window of an A/P enhancer is a 960 bp sequence centred around the Bicoid-binding site cluster. Each orthologous set of NEEs is boxed separately to visualize enrichment relative to other groups. The red boxes show the regions occupied by all data points corresponding to a single orthologous set of NEEs located at the indicated locus across many species. The blue box shows the region occupied by all data points corresponding to all A/P enhancers for all species. ( b ) Identical graph as in panel a , except the data points are boxed by species to visualize genome-specific effects in satellite enrichment or depletion. Red boxes show the region occupied by all data points corresponding to all NEEs within a single species. Canonical A/P enhancers at the eve , gt , Kr and hb loci for all four species are boxed in both panels (blue rectangular area). ( c ) Graph showing the number of cells spanned by the lacZ expression pattern (vertical axis), as driven by NEEs containing different numbers of Dl half-sites, 5′-SGGAAW-3′ (horizontal axis). ( d ) Graph showing the number of cells spanned by the lacZ expression pattern (vertical axis), as driven by NEEs characterized by different E-to-D spacer lengths (horizontal axis). Error bars in c and d represent ±1 s.d., as derived from a replicate pool of 20–120 embryos for each construct. Full size image We then investigated the relation between threshold readout and the density of Dl half-sites in a region anchored ±480 bp from D β ( Fig. 5c ). Despite using diverse descriptors of a Dl site, we find no relation between Dl-binding site densities and stripe width measured at 50% egg length. Identical densities of Dl half-sites, degenerate full-sites and more complete full-sites are present in different enhancers that readout different Dl concentration thresholds and vice versa. In contrast, if we plot the length of threshold spacers for different NEEs from different species, except those from the dorsally repressed vnd loci, we see a well-defined, hump-shaped curve, whose peak activity tops at around ∼ 8 to 12 bp and falls on either side of this maximum ( Fig. 5d ). The spacer elements from the consistently high-threshold NEE vnd sequences obey a similar, although depressed, curve across the genus because of one additional regulatory input, which we will describe in a future study. Thus, there is a tremendous sequence bias that is unique to canonical NEEs across the genus. Although non-functional, this compositional bias is related to specific threshold setting elements employed by NEEs. This suggests that the frequency of threshold replacement during lineage evolution is high. Dl relic elements bias site sequence selection A high frequency of threshold replacement suggests that the specialized SUH / D α site may originate as a D β relic element that is exapted into a Su(H)-binding site. We therefore compared the D α and D β consensi motifs across all five divergent Drosophila lineages for which we functionally tested NEEs ( Fig. 6a ). We find that the first half of the D α motif, which overlaps the Su(H)-binding motif, is conserved whereas the second half is increasingly degenerate relative to the inferred ancestral D α motif, which resembles a D β motif itself (compare Su(H) with D α motifs in Fig. 6a ). 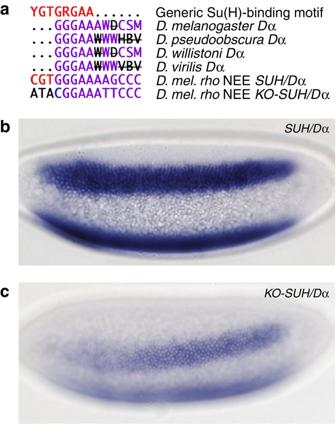Figure 6: Su(H)-binding sites are exapted from Dl relic sequences in mature NEEs. (a) Alignment of the lineage-specific consensi forDα shows that the portion overlapping the Su(H)-binding site is the least divergent (purple), whereas the second half-site is degenerate relative to other lineages (black struck-out letters). Also shown are the wild-type and mutated sequences of this site tested in therhoNEE fromD. melanogaster(D. mel.). (b,c) TypicallacZexpression patterns driven byrhoNEE reporters containing the fullSUH/Dα site (b) or the knocked out (KO) Su(H) site (c). Figure 6: Su(H)-binding sites are exapted from Dl relic sequences in mature NEEs. ( a ) Alignment of the lineage-specific consensi for D α shows that the portion overlapping the Su(H)-binding site is the least divergent (purple), whereas the second half-site is degenerate relative to other lineages (black struck-out letters). Also shown are the wild-type and mutated sequences of this site tested in the rho NEE from D. melanogaster ( D. mel. ). ( b , c ) Typical lacZ expression patterns driven by rho NEE reporters containing the full SUH / D α site ( b ) or the knocked out (KO) Su(H) site ( c ). Full size image To test whether the Su(H)-binding site is itself functional and perhaps the principal reason for persistence of a 'ghost' D α motif, we knocked out the Su(H)-specific portion of the SUH / D α site in the NEE rho sequence of D. melanogaster and tested this modified enhancer in our standard transgenic reporter assay (see KO-SUH in Fig. 6a ). We find that this mutation weakens the activation response of the enhancer without affecting the specific threshold setting ( Fig. 6b–c ). We suggest that runaway CA-satellite expansions in relic E(CA)T sequences push coordinating Su(H)-binding elements away from active E-to-D encodings, and that this engenders selection for closer Su(H)-binding sites in aging NEEs. Consequently, because mature NEEs contain deprecated D β relic sites, whose palindromic half-sites resemble the last six nucleotides of a generic Su(H)-binding motif (5′-YGT GRGAAM -3′), closer Su(H)-binding sites are exapted from Dl relic sites. Newly evolved NEEs are not enriched in relic sites Our model of threshold evolution suggests that NEE signatures are missed in whole-genome bioinformatic searches that use overly determined SUH / D α motifs. We documented a lineage-specific NEE sequence at the sog locus of D. melanogaster [6] , but because the CA content of NEEs from D. melanogaster may have been secondarily reduced during genome compaction, we sought to identify recently evolved NEEs from larger genomes for unambiguous interpretation. We therefore searched the two largest Drosophila genome assemblies, which correspond to D. ananassae (231.0 Mb) and D. willistoni (235.5 Mb). Of the 1 kb genomic windows centred on all D β sequences in any given genome and containing E(CA)T anywhere in that window, we identified those sequences that contain an E-to - D encoding and an 8 bp degenerate Su(H)-binding motif (5′-YGYGRGAA-3′) instead of the 14 bp SUH / D α motif. Using this set of minimal criteria, we identified the canonical NEE repertoires in each species and one additional positive hit in D. ananassae . From the D. ananassae genome, we cloned and assayed both a functional set of canonical NEEs ( Fig. 7a–d ) and a new NEE at the Delta locus ( Fig. 7e–f ). Delta encodes a ligand for the Notch receptor, whose signalling is relayed by Su(H) [47] , [48] . In D. melanogaster embryos, Delta is expressed in a narrow lateral stripe in the mesectoderm and ventral-most row of the neurogenic ectoderm using sequences that are unrelated to the unique NEE Delta sequence of D. ananassae [49] . This NEE Delta sequence has not acquired either CA-satellite fragments or Dl relic sequences ( Fig. 7e ). Nonetheless, this enhancer is functional in D. melanogaster embryos ( Fig. 7f ). Furthermore, its Su(H)-binding site does not overlap the ghost D α motif that characterizes the canonical NEEs of the genus ( Fig. 7g ). Altogether, our data on the NEE Delta sequence suggest a shorter period of evolutionary maintenance, as is consistent with its more recent phylogenetic origin relative to canonical NEEs. 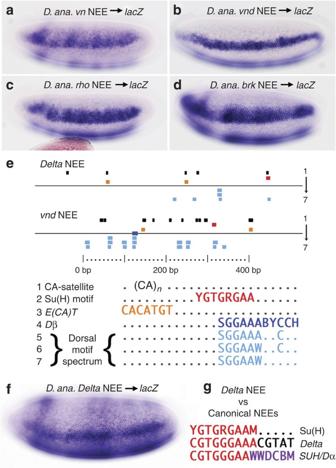Figure 7: Recently evolved NEEs have not accumulated relic element clusters. (a–d) NEE-drivenlacZ in situhybridization experiments forD. ananassae(D. ana.) NEEs. Shown are lateral stripe expression patterns that are typical of multiple transgenicD. melanogasterlines made with theD. ananassaeNEEs fromvn(a),vnd(b),rho(c) andbrk(d). (e) Diagram of relic site clusters for theDeltaandvndNEEs fromD. ananassae. Matches to CA satellite on either strand (black), Su(H)-binding motif (red),E(CA)T(orange),Dβ (dark blue) and aDβ motif spectrum (light blue) are visualized in separate numbered tracks (1–7) at the top and described in more detail below. CA satellite is defined here as sequences matching two CA-dinucleotide repeats or longer given by the perl regular expression: 'A?(CA){2,}C?'. (f) The typicallacZ in situhybridization experiment forD. ananassae DeltaNEE. (g) A comparison of theDeltaNEE Su(H)-binding site and downstream flanking sequence and theDα motif forD. ananassae. The flanking sequence at theDeltasite (black lettering) is unrelated to a Dl half-site. Figure 7: Recently evolved NEEs have not accumulated relic element clusters. ( a – d ) NEE-driven lacZ in situ hybridization experiments for D. ananassae ( D. ana. ) NEEs. Shown are lateral stripe expression patterns that are typical of multiple transgenic D. melanogaster lines made with the D. ananassae NEEs from vn ( a ), vnd ( b ), rho ( c ) and brk ( d ). ( e ) Diagram of relic site clusters for the Delta and vnd NEEs from D. ananassae . Matches to CA satellite on either strand (black), Su(H)-binding motif (red), E(CA)T (orange), D β (dark blue) and a D β motif spectrum (light blue) are visualized in separate numbered tracks (1–7) at the top and described in more detail below. CA satellite is defined here as sequences matching two CA-dinucleotide repeats or longer given by the perl regular expression: 'A?(CA){2,}C?'. ( f ) The typical lacZ in situ hybridization experiment for D. ananassae Delta NEE. ( g ) A comparison of the Delta NEE Su(H)-binding site and downstream flanking sequence and the D α motif for D. ananassae . The flanking sequence at the Delta site (black lettering) is unrelated to a Dl half-site. Full size image To understand the origin of complex homotypic site clusters in relation to the Dl morphogen concentration threshold-encoding scheme of NEEs, we conducted a comparative study of such sequences isolated from Drosophila species with the largest sequenced genomes. Our results support a novel evolutionary model that describes how selective maintenance of optimal threshold encoding results in complex non-functional sequence signatures over time ( Fig. 8 ). 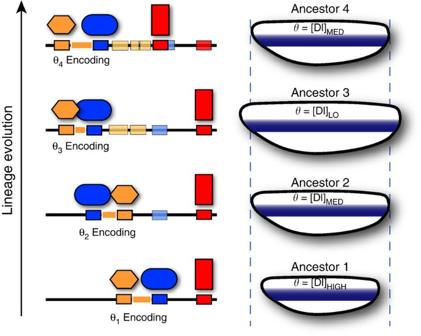Figure 8: Evolutionary origin of relic element clusters. On the left are diagrams of an evolving NEE configuration and on the right are hypothetical embryos of evolving size, which necessitate the implementation of different concentration thresholds (high (HIGH), medium, (MED), low (LO) and medium (MED)) by the enhancer (indicated by indexed theta symbols). The ancestral NEE configuration is depicted at the bottom and increasingly more recent configurations are depicted above the earlier configurations. Other potential reasons for threshold evolution are possible but are not shown. In the NEE site configurations, Dl- and Twi-binding sites are depicted by blue and orange boxes, respectively, and their relic counterparts in similar but more transparent boxes. Su(H)-binding sites are depicted in red boxes. Transcription factor proteins that recognize the functional elements are also indicated. Figure 8: Evolutionary origin of relic element clusters. On the left are diagrams of an evolving NEE configuration and on the right are hypothetical embryos of evolving size, which necessitate the implementation of different concentration thresholds (high (HIGH), medium, (MED), low (LO) and medium (MED)) by the enhancer (indicated by indexed theta symbols). The ancestral NEE configuration is depicted at the bottom and increasingly more recent configurations are depicted above the earlier configurations. Other potential reasons for threshold evolution are possible but are not shown. In the NEE site configurations, Dl- and Twi-binding sites are depicted by blue and orange boxes, respectively, and their relic counterparts in similar but more transparent boxes. Su(H)-binding sites are depicted in red boxes. Transcription factor proteins that recognize the functional elements are also indicated. Full size image NEEs encode a specific concentration threshold response by containing a single E-to-D threshold-encoding sequence near a Su(H)-binding site (bottom of Fig. 8 ). An E-to-D encoding functionally maps a DNA spacer length of 3–15 bp, which separates a pair of well-defined Dl- and Twi-binding elements, onto one well-defined dorsal border of expression that is 5–15 nuclei past the ventral border of the neurogenic ectoderm. Certain features that are inherent to E-to-D encodings facilitate the selection for changes in threshold through simple mutational alterations. The foremost feature is that the Twi-binding site can occur in the form of a CA-satellite-rich sequence that is prone to repeat expansions and contractions that can redefine the spacer length and threshold setting. Consequently, this E(CA)T instability becomes the mutational source of all new threshold variants. Second, because the Dl- and Twi-binding sites are palindromes, threshold evolution may proceed through selection of one new site adjacent to an E-to-D encoding (see leap-frogging of sites during evolution of thresholds from θ 1 to θ 2 , and again from θ 2 to θ 3 in Fig. 8 ). Such a new site can define a new spacer length and threshold setting. This evolutionary process of threshold selection readily produces eclipsed Dl- and Twi-binding elements that decay as relic elements. Third, the broad functional range of E-to-D encodings increases the number of possible variants with incrementally optimized thresholds. Our data suggest that relic element accumulation begins with each NEE origination and is continuously co-extant with its adaptive maintenance. With increasing time, the background sequence composition of enhancers is profoundly altered and eventually dominates the nature of binding site selection because it provides a highly biased ground state from which new sites are exapted (top of Fig. 8 ). In principle, plaques of relic elements will accumulate in complex eukaryotic enhancers that encode threshold response variables in a precise syntax that is under constantly shifting selection. Regulatory evolution may underlie many of the stabilizing and adaptive changes associated with both normal lineage persistence and event-driven originations of new lineages. During such scenarios, the potential for gene regulatory evolution is facilitated by DNA regulatory systems that encode broad-ranged response variables. However, a broad or evolutionarily varied phenotypic range may be an indirect consequence of molecular mechanisms that are employed ontogenetically at multiple loci in precise but functionally varied configurations, as we have documented. In this regard, we point out that the Dl–Twi protein complex assembling on NEEs appears to be functioning as a pair of molecular calipers for measuring the precise lengths of DNA at different enhancers. Several interesting lines of questioning present themselves and we hope we can address these with protein biochemistry conducted in the context of informative configurations of key DNA sequences. Embryonic experiments Animal rearing, P-element-mediated transformations, embryonic collections, staging, anti-DigU probe synthesis and whole-mount in situ hybridizations were conducted on stage 3 to stage 6 embryos that were dechorionated, devitellizied, fixed in formaldehyde and dehydrated in EtOH [6] . D. willistoni and D. ananassae strains were obtained from stock centres and reared at ∼ 23 °C (room temperature) using standard D. melanogaster media. Probes for whole-mount in situ hybridization in D. willistoni embryos Primers for probe synthesis are as listed here. rho : 5′-CCGCCTTTGCCTATGACCGTTATACAATGC-3′ and 5′-Pr-TTAGGACACACCCAAGTCGTGC-3′, where Pr = the T7 promoter sequence 5′-CCGCCTAATACGACTCACTATAGGG-3′. vn : 5′-CCGCCTAGTGACGACAACAACAACAGTAGC-3′ and 5′-Pr-ATTTTCACTCACAGCCATTTTCACC-3′. vnd : 5′-CCGCCCTAGTCCGGATAGCACTTCGC-3′ and 5′-Pr-CGGCTGCCACATGTTGATAGG-3′. brk : 5′-CCGCCAACAAAGTTCGTCGGCAACAACG-3′ and 5′-Pr-CATGGTGAGGTGAGGACTATGG-3′. Whole-genome sequence analysis Current versions for all genomes were downloaded from Flybase ( http://www.flybase.org ) and these correspond to assembly versions: dmel ver5.22, dana ver1.3, dpse. ver2.6, dwil ver1.3 and dvir ver1.2. We wrote UNIX-shell script programs that employ grep and perl programs. We used these script programs on FASTA genome assembly files (for example, 'dmel-r5.22.txt') to produce a HEADER-FREE, N-FREE, fly genome file, indicated by the file extension '.HNF'. We used these files to identify and count substrings without counting N's and header characters. This script also produces the '.ONE' file from the '.HNF' file. The '.ONE' file has no newlines and can be used to count known nucleotides without counting newlines using the UNIX command 'wm -m dmel-r5.22.ONE'. The '.HNF' files are processed by an additional script to identify a substring, remove newlines and count characters and so on. All script and sequence files are provided in two b-zipped, archived Supplementary Software files corresponding to NEE composition and CA-satellite analyses. How to cite this article: Justin C., et al . Dynamic evolution of precise regulatory encodings creates the clustered site signature of enhancers. Nat. Commun. 1:99 doi: 10.1038/ncomms1102 (2010).